Supramolecular catalysis with ethers enabled by dual chalcogen bonding activation 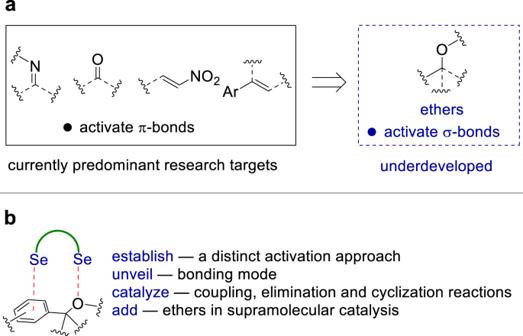Fig. 1: Catalysis with weak interactions. aAn overview on catalysis with weak interactions.bThis work: supramolecular catalysis with ethers. The activation of ethers by weak interactions is a long-standing objective in supramolecular catalysis, but yet it remains an underdeveloped topic. The obstacles towards solving this problem are prominent since it is difficult for a weak interaction to cleave a relatively strong C-O σ-bond and moreover, the ionic intermediate composing of an alkoxide ion and an electrophilic carbocation would deactivate weak interaction donors. Herein, we describe a distinctive activation mode, dual Se···π and Se···O bonding, that could activate benzylic as well as allylic ether C-O σ-bonds to achieve cyclization, coupling and elimination reactions. This dual Se···π and Se···O bonding catalysis approach could tolerate various alkoxide leaving groups, while the other representative weak interaction donors showed no catalytic activity. Catalysis with weak interactions has been established as a fundamental discipline in organic synthesis [1] . A large number of chemical transformations were achieved by hydrogen bonding interactions [2] as well as the lately established catalysis modes such as halogen [3] , [4] , [5] , [6] , chalcogen [5] , [6] , [7] , [8] , [9] , [10] and carbon bonding [11] interactions. Generally, the success of this research area relies on the activation of comparatively reactive π‒bonded functional groups, with carbonyl, imine, and nitro groups as dominant targets (Fig. 1a ) [1] .It has been generally considered that it is difficult to weaken a strong σ‒bond to generate reactivity by imposing of weak interactions on an organic molecule [1] , [2] , [3] , [4] , [5] , [6] , [7] , [8] , [9] , [10] , [11] , [12] . Accordingly, the catalytic activation of relatively strong σ‒bonds by weak interactions has been recognized as a long-standing challenge in supramolecular catalysis [1] , [2] , [3] , [4] , [5] , [6] , [7] , [8] , [9] , [10] , [11] , [12] . In this context, research toward solving this severe limitation emerges as an urgent and essential goal. Fig. 1: Catalysis with weak interactions. a An overview on catalysis with weak interactions. b This work: supramolecular catalysis with ethers. Full size image As a representative case, even though benzylic as well as allylic ethers are frequently used reactants in organic synthesis, the activation of these ethers is not trivial. Generally, metal catalysts, superacid or strong photochemical conditions were employed to activate benzylic and allylic ethers [13] , [14] , [15] , [16] , [17] , [18] , [19] . Owing to the relatively strong C-O σ-bonds and the intractable alkoxide leaving group [20] , it appears rather difficult for a metal-free approach to activate ethers, for instance, the coupling reactions between benzylic ethers and electron rich arenes requires the use of a stoichiometric amount of superacid BF 3 –H 2 O and a high temperature (120 °C) [13] . In this context, the practices in supramolecular catalysis suggest the activation of ethers by weak interactions is an unfavorable approach [1] , [2] , [3] , [4] , [5] , [6] , [7] , [8] , [9] , [10] , [11] , [12] , and it remains an underexplored topic (Fig. 1a ). Apparently, the comparatively strong C‒O σ‒bond sets up a hard-to-reach barrier for weak interactions to play an effective role in activating ethers [12] . Moreover, even supposing that the cleavage of an ether C‒O σ‒bond by a weak interaction is possible, the ionic intermediate is constituted by two problematic species, a strongly alkaline and nucleophilic alkoxide and an electrophilic carbocation, which would potentially deactivate weak interaction donors by routine approaches such as competitive bonding, deprotonation, nucleophilic/electrophilic substitutions. Despite these glaring problems, however, the activation of ethers by weak interactions would serve as an important step for weak interactions to enter an area dealing with relatively strong σ-bonds. Recently, contrary to the conventional covalent Lewis base property [21] , disubstituted chalcogens that bear two lone pairs were used as electron acceptors to operate noncovalent chalcogen bonding interactions, which have been found applications in a broad chemical context including drug discovery, material chemistry, crystal engineering, anion recognition, and controlling of the conformations of reaction intermediates [22] , [23] , [24] , [25] , [26] , [27] , [28] , [29] , [30] , [31] . Several disubstituted chalcogens were used as chalcogen bonding catalysts, such as dithieno[3,2-b;2’,3’-d]thiophenes [32] , [33] , bis(benzimidazolium) chalcogenides [34] , [35] , [36] , [37] , [38] , and phosphonium chalcogenides [39] , [40] , [41] , [42] , [43] . To add ethers in the list of supramolecular catalysis, herein, we unveil a dual Se···π and Se···O bonding mode for the activation of ethers, and demonstrate its application in catalytic cyclization, coupling, elimination and the Friedel-Crafts reactions (Fig. 1b ). Considering the substantial difference between the strong covalent activation and the weak interaction approaches, the dual chalcogen bonding catalysis approach has its unique advantage, which proceeds in the absence of any metal additive while it can give reactivity and enhance the reaction selectivity. Chalcogen bonding interactions Initially, judging by the reported precedents in supramolecular catalysis [1] , we were unaware that the weak strength of chalcogen bonding interactions would be capable of activating ether C-O σ-bonds. On the other hand, it was observed that the use of an ether solvent often resulted in an inhibition of reactions to some extent [41] , indicating the presence of competitive chalcogen bonding between substrate and ether solvent. In this context, an investigation on chalcogen bonding interactions between selenides and ethers was carried out (Fig. 2 ). To this end, a representative chalcogen bonding donor Ch1 was chosen as an optimal target to study chalcogen bonding interactions (Fig. 2a ). Analysis of a 1:1 mixture of Ch1 and ether e1 in CD 2 Cl 2 by 13 C NMR revealed that there is almost no variation of the 13 C signals of e1 (for all carbons <0.05 ppm). Similar results were obtained using selenide Ch2 , since almost no variation of the 13 C signals of e1 (for all carbons <0.05 ppm) was observed, even in the presence of a 2:1 mixture of Ch2 : e1 . Fig. 2: Chalcogen bonding interaction with ethers (concentration: 0.10 M −1 for bidentate donor; 0.10 M −1 for ether; 0.20 M −1 for monodentate donor). a The interaction between chalcogen bonding donors and e1 . b The interaction modes between chalcogen bonding donors and ethers. c The match and mismatch of binding sites between chalcogen bonding donors and ethers. d Molecular control experiments. BAr F 4 ‾: tetrakis[3,5-bis (trifluoromethyl)phenyl]borate. Full size image In contrast, however, analysis of a 1:1 mixture of Ch3 and e1 in CD 2 Cl 2 by 13 C NMR shows that the 13 C signal of the carbon (C Bn ) attached to oxygen shifts downfield by 0.12 ppm. A much more dramatic variation of the chemical shift of 13 C signals arises from the phenyl ring. The aromatic carbon C a shifts upfield as much as −0.48 ppm while the other aromatic carbons (C b ‒C d ) shifts downfield from a range of 0.08 to 0.21 ppm. For comparison, the monodentate counterpart of Ch3 , i.e. Ch4 , was investigated. Analysis of a 2:1 mixture of Ch4 : e1 in CD 2 Cl 2 by 13 C NMR reveals that there is almost no perturbation of the 13 C signals of e1 . To explain these experimental results, several possible bonding modes were depicted in Fig. 2b . The performance of monodentate Ch2 and Ch4 indicates a single interaction mode COM1 or COM2 is not productive. Meanwhile, the sharp contrast between Ch3 and its monodentate counterpart Ch4 indicates a dual interaction mode is in operation. In addition, the variation of the 13 C signals was observed not only from the carbon attached to oxygen of e1 but more marked perturbation from the remote aromatic ring. These results suggest that a dual Se···π and Se···O bonding mode ( COM3 ) is likely the operative one, while they are against mode COM4 . In addition, since chalcogen bonding is almost a linear interaction [12] , it is unfavorable to form COM4 upon considering the bonding angles of Ch3 . To enable a dual Se···O and Se···π bonding mode COM3 , a good match of the bonding sites between an ether and a chalcogen bonding donor is essential (Fig. 2c ). The interaction of Ch3 with different ether showed that the perturbation of the chemical shift of 13 C signals of phenyl ring decreased dramatically upon increasing the distance between the oxygen atom and phenyl ring in ethers e1 - e3 (0.48, 0.23 and 0.14 ppm corresponding to C a of e1 , e2 , e3 ). Alternatively, upon maintaining ether e1 unchanged, the increasing of the distance between two selenium atom leads to a decreased variation of the chemical shift of 13 C signals. In the presence of Ch5 and Ch6 , only 0.09 and 0.05 ppm change of C a in e1 were observed. Upon further increasing the chain length, bidentate Ch7 performs like a monodentate selenide. The steric hindrance arising from the substitutions of phenyl ring in a modified e1 could block the Se···π interaction to some extent, thus resulting in a less marked variation of 13 C signals of phenyl ring. To investigate Se···π interaction, three isopropyl groups were installed in the phenyl ring of e1 to give a reference ether e4 . The experimental result is in line with this notion, and a smaller variation (i.e. 0.24 vs 0.48 ppm) of the 13 C signal of C a of e4 was observed (Fig. 2d ). In addition, an intramolecular competition experiment was carried out to corroborate the Se···π interaction. To this end, two aromatic rings with distinct steric hindrance were installed in ether e5 (i.e. i -Pr 3 Ph vs Ph). The experiment results showed that the 13 C signal of C a ’ in Ph varies 0.16 ppm, while a decreased perturbation of its steric counterpart C a in i -Pr 3 Ph (−0.03 ppm) was obtained. In contrast, the variation of both the 13 C signals of C a ’ and C a in e6 could be observed. These molecular control experiments further support a bonding mode of COM3 . The Se···O interaction would polarize the C-O bond to facilitate the heterolytic cleavage. On the other hand, the Se···π bonding leads to a distinct shift of the 13 C signals of the aromatic ring. Using e1 as an example, the 13 C signal of aromatic carbon C a attached to benzylic carbon shifts upfield dramatically (−0.48 ppm), while the 13 C signals of the other aromatic carbons (C b ‒C d ) shift downfield (+0.08 to +0.21 ppm). Since C a is attached to the benzylic carbon, the above observation could be rationalized by electron‒withdrawing via Se···π bonding which lowers the π* energy, thus leading to an increased σ→π* charge transfer. As a result, a marked shielding of C a was observed owing to an increased electron density of C a , which in turn contributes to the cleavage of C‒O bond. To understand the chalcogen bonding interaction with ether, density functional theory (DFT) calculations were carried out at M06-2X/6-311 g(d,p) level of theory corrected with the Grimme’s dispersion (D3) [44] . The electrostatic potential map in Fig. 3a suggests that the two selenium atoms have highly electropositive sites and the electrostatic potential values are +114.6 and +116.1 kcal/mol, respectively. As shown in Fig. 3b , in contrast to the Se···O bonding complex COM1 , the results of DFT calculations suggest that an additional Se···π interaction in COM3 could significantly lower the energy barrier to generate the selenide-ether bonding complex. Further NCI analysis in Fig. 3c shows main noncovalent interactions. Light blue regions representing relatively strong interactions between Se···O exist in both the complexes of COM1 and COM3 , indicating that Se···O interactions contribute significantly to the formation of these supramolecules. While π···π interaction could be observed in COM1 , the computational results suggest it is more favarouble to generate COM3 owing to the contribution of Se···π interaction. Fig. 3: DFT calculations. a Electrostatic potential map. b Optimized complexes. c NCI analysis of complexes. Full size image In principle, the increasing of the concentration of ether e1 results in the generation of a higher concentration of equilibrating supramolecular bonding complexes. The donation of electron from ether to selenium would change the electron distribution around selenium, thus potentially having an effect on the spin-spin coupling. A significant observation is that the concentration of ether e1 has a correlation with the variation of coupling constant 1 J P,Se (Fig. 4 ). A general trend is that a higher concentration of e1 resulted in a more dramatic variation of the coupling constant. In the presence of 2.0 M e1 , the coupling constant 1 J P,Se varies as much as 2.2 Hz in contrast to Ch3 itself. Fig. 4: The variation of coupling constant. Relationship between the coupling constant of 1 J P,Se of Ch3 and the concentration of e1 . Full size image To provide some information on the chalcogen bonding between selenide and ether, chalcogen bonding donor Ch8 bearing a benzylic ether fragment was synthesized (Fig. 5 ). The X-ray crystal structure of Ch8 shows the presence of an intramolecular Se···O interaction, wherein the distance between Se and O is 2.77 Å which is markedly shorter than the sum of their van der Waals radii 3.42 Å while the interaction angle of C-Se···O is 165.3˚. For intermolecular interactions, Se···π bonding interactions are more favorable than Se···O interactions in the packing diagram of Ch8 . Fig. 5: Structure and bonding. Intramolecular Se···O and intermolecular Se···π interactions in the crystal structure of Ch8 ; Intra- and intermolecular Se···π interactions in the crystal structure of Ch9 ; Intermolecular Se···O interactions in the cocrystal structure of Ch5 and dioxane. Hydrogens and counteranions were omitted in these X-ray crystal structures for clarity. Full size image To further unveil the intermolecular Se···π bonding interaction, the less coordinating BAr F 4 ‾ counteranion in Ch3 was replaced by triflimide, i.e. (CF 3 SO 2 ) 2 N‾ (Fig. 5 ). Despite the presence of multiple oxygen binding sites in counteranion, the crystal structure of Ch9 shows that the intermolecular interactions were dominated by Se···π bonding interactions. On the other hand, the co-crystal structure of Ch5 and 1,4-dioxane shows the presence of a bonding complex operated through the intermolecular Se···O interactions (Fig. 5 ). These crystal structures depicted in Fig. 5 suggest it is possible for this type of selenides to interact with an ether to form Se···O and Se···π bonding interactions. Supramolecular catalysis with ethers For the activation of benzylic ethers, the observations in Fig. 2 suggest that (1) bidentate Ch3 is more efficient than the other counterparts, and (2) monodentate Ch2, 4 and bidentate Ch1 with a rigid backbone, which are difficult to interact with both the oxygen atom and the phenyl ring in ether simultaneously, are not productive. Furthermore, bidentate selenides Ch5 - 7 with a longer linker are less effective. To verify such a relationship between the structure and catalytic activity, the Friedel-Crafts reaction between ether 1a and m -xylene 2a was employed (Fig. 6 ) [13] , [14] , [15] , [16] , [17] , [18] . In the absence of a promoter, the reaction between 1a and 2a did not take place. In line with the above observations, catalyst Ch1 was inactive in this reaction, while Ch3 gave the best results among these catalysts. Accordingly, catalysts Ch2 / 4 showed no or low catalytic activity (Fig. 6 ). The catalytic activity decreased gradually upon increasing the length of linker from one carbon to eight carbons ( Ch5 - 7 ). Fig. 6: Structure and catalytic activity. Distinct catalytic activity for chalcogenides Ch1 - 7 . Catalytic performance for reference hydrogen- and halogen-bonding catalysts H1 , H2 and XB . DCE: 1, 2-dichloroethane. Full size image Tracing the reaction system by 31 P NMR indicated that catalyst Ch3 was stable under this reaction condition and only 31 P signal corresponding to Ch3 was observed (see Supplementary Fig. 11 ). For reference, the other types of weak interaction donors were investigated (Fig. 6 ). The experimental results showed that the representative hydrogen bonding catalysts H1 - 2 and halogen bonding catalyst XB , had no catalytic activity. Furthermore, this reaction did not work in the presence of 10 mol % TsOH or CF 3 COOH even at 50 o C. The strength of chalcogen bonding interactions follows the order of S < Se [45] . Accordingly, a decreased catalytic activity in principle would be expected upon replacement of the selenium atom in Ch3 with sulfur (Fig. 7a ). In line with this notion, the experimental results indicated that sulfur-based donor Ch10 gave a lower catalytic activity in contrast to Ch3 . On the other hand, since S is more electronegative than Se, phosphorus part in Ch10 is therefore more positively charged than that in Ch3 , which is consistent with the results of 31 P NMR experiments (42.30 ppm for Ch10 vs 30.27 ppm for Ch3 ). Taking the structure and catalytic performance into consideration, the comparison between Ch10 and Ch3 suggests that the catalytic activity arises from the selenium part. Fig. 7: Structure and catalytic activity. a Comparing the catalytic activity of analogous catalysts Ch3 , Ch10 , and Ch11 . b Catalytic activity of reference catalysts Ch12 - 15 . Full size image Since chalcogen bonding is a type of highly directional interaction, the steric hindrance of the selenium part could prevent the electron donors to approach selenium, thus deactivating the catalyst to some extent. Then a more steric catalyst Ch11 was synthesized. In agreement with the chalcogen bonding property, the installation of isopropyl groups in the phenyl ring attached to selenium of Ch3 led to a decreased catalytic activity (Fig. 7a ). To provide further information, monodentate catalysts Ch12 and Ch13 was synthesized, and they showed no catalytic activity (Fig. 7b ). The distinct catalytic activity of bidentate catalyst Ch3 and these monodentate catalysts underscores the importance of a dual interaction. Further investigation using catalyst Ch14 suggests that the attachment of a phenyl group to selenium is not essential since a methyl group attached to selenium was catalytically active, and product 3 was obtained in 41% yield (Fig. 7b ). We further tested one of the most active catalysts that we have ever obtained, i.e. catalyst Ch15 [43] . Because Ch15 could not interact with benzylic ether via a dual interaction approach, it showed no catalytic activity (Fig. 7b ). These additional results indicate the essential role of a dual activation approach. The experimental results showed that a diverse array of alkoxide ions including MeOˉ, BnOˉ, PhOˉ and n -PrOˉ could serve as effective leaving groups (Fig. 8a ). For substrate 1c , the 13 C NMR analysis of 1:1 mixture of 1c and Ch3 in CD 2 Cl 2 revealed that the perturbation of the 13 C signals is similar upon comparing the two phenyl rings of 1c . For this chalcogen bonding catalysis approach, the complexation of catalyst and ether is an essential process but is not the rate-determining step. Once the supramolecular bonding complex is formed, the more favorable C-O bond cleavage enabling the formation of a more stable carbocation determines the reaction outcome. Moreover, a range of siloxides such as Me 3 SiOˉ, t -BuMe 2 SiOˉ and t -BuPh 2 SiOˉ were also demonstrated to be effective leaving groups. For substrate 1 g , phenol would be generated along with the desirable product 5 , which could in turn competitively react with ether 1 g to give a side product ( vide infra , compound 19 ). Further investigation revealed that both benzylic and allylic ethers could be activated to participate in different reaction processes, giving products 6-22 in moderate to good yields (Fig. 8b ). Upon addition of 1.0 equiv CaH 2 to the catalysis system, product 6 was obtained in 76% yield and the reaction efficiency was not affected. Furthermore, this reaction did not work in the presence of 10 mol % TsOH or CF 3 COOH. For products 8 and 19 , their ortho-selective regioisomers were obtained in 14% and 16% yields, and the isomeric ratios are 1:4.6 and 1:4.2, respectively. Fig. 8: Chalcogen bonding catalytic transformation of ethers. a Alkoxide leaving groups. b Coupling reactions. Full size image Generally, alkoxide ions are considered as poor leaving groups to engage in elimination reactions. Instead of trapping with a nucleophile, the in situ generated carbocation could undergo an elimination process. This dual Se···O and Se···π bonding activation approach enables elimination reaction of ether to take place in a highly stereoselective manner. As shown in Fig. 9 , a controlled synthesis of specific stereoisomer could be achieved using this method, and the elimination of ether 1 u gave product ( E )- 23 in 76% yield with 14.5:1 E / Z stereoselectivity. In contrast, a metal Lewis acid approach, i.e. FeCl 3 , afforded lower selectivity ( E / Z 8.2:1) in 79% yield. Fig. 9: Stereospecific elimination. Chalcogen bonding catalysis approach to the elimination of ether 1 u . The use of FeCl 3 as a reference Lewis acid catalyst for the elimination of ether 1 u . Full size image Using Boc-protected pyrrolidine derivative 1 v as a reactant, an intramolecular cyclization reaction took place to give heterocycle 24 in 71% yield (Fig. 10a ). Upon replacement of TMS with Me, substate 1w underwent the same cyclization reaction to give product 24 in 73% yield. Furthermore, under catalysis of Ch3 , a cyclization reaction took place and ether 1x was directly transformed to product 25 (Fig. 10b ). Upon addition of either 1.0 equiv K 2 CO 3 or CaH 2 to the catalysis system, the reaction proceeded with almost the same efficiency, and product 25 was obtained in 71% and 69% yields, respectively. Furthermore, tracing this reaction system by 31 P NMR revealed that catalyst Ch3 remained unchanged since only 31 P signal corresponding to Ch3 was observed (see Supplementary Fig. 13 ). Fig. 10: Cyclization of ethers. 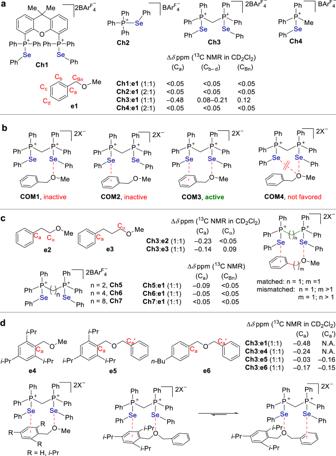Fig. 2: Chalcogen bonding interaction with ethers (concentration: 0.10 M−1for bidentate donor; 0.10 M−1for ether; 0.20 M−1for monodentate donor). aThe interaction between chalcogen bonding donors ande1.bThe interaction modes between chalcogen bonding donors and ethers.cThe match and mismatch of binding sites between chalcogen bonding donors and ethers.dMolecular control experiments. BArF4‾: tetrakis[3,5-bis (trifluoromethyl)phenyl]borate. a Intramolecular cyclization reactions of 1 v and 1w . b Intermolecular cyclization reaction of 1x . Full size image In conclusion, this work demonstrates that a rationally designed weak interaction mode is capable of activating relatively strong C-O σ-bonds of ethers, which is of vital importance for a sustainable development of supramolecular catalysis. 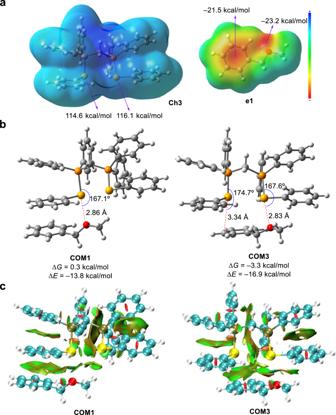Fig. 3: DFT calculations. aElectrostatic potential map.bOptimized complexes.cNCI analysis of complexes. The experimental results suggest a dual Se···π and Se···O bonding mode is in operation for the activation of benzylic as well as allylic ethers. 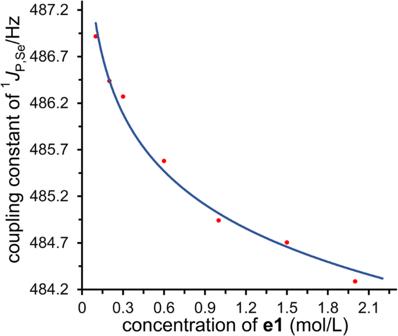Fig. 4: The variation of coupling constant. Relationship between the coupling constant of1JP,SeofCh3and the concentration ofe1. This catalysis mode could be applied to a diverse array of transformations including coupling, elimination, cyclization and the Friedel-Crafts reactions, thus enabling adding ethers in the list of supramolecular catalysis. General procedure for chalcogen bonding catalytic transformation of ethers To a reaction mixture of catalyst Ch3 (10 mol %, 0.02 mmol) in a 10 mL-Schlenk tube was added DCE (1.0 mL) under argon atmosphere. Then ether substrate 1 (0.2 mmol) and nucleophile (0.6 mmol, 3.0 equiv) was added to the above reaction mixture. 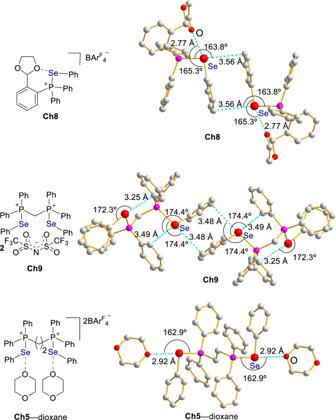Fig. 5: Structure and bonding. Intramolecular Se···O and intermolecular Se···π interactions in the crystal structure ofCh8; Intra- and intermolecular Se···π interactions in the crystal structure ofCh9; Intermolecular Se···O interactions in the cocrystal structure ofCh5and dioxane. Hydrogens and counteranions were omitted in these X-ray crystal structures for clarity. The reaction was stirred at room temperature until the completion of the reaction as judged by TLC analysis. 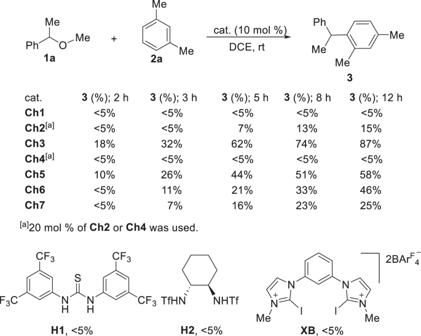Fig. 6: Structure and catalytic activity. Distinct catalytic activity for chalcogenidesCh1-7. Catalytic performance for reference hydrogen- and halogen-bonding catalystsH1,H2andXB. DCE: 1, 2-dichloroethane. 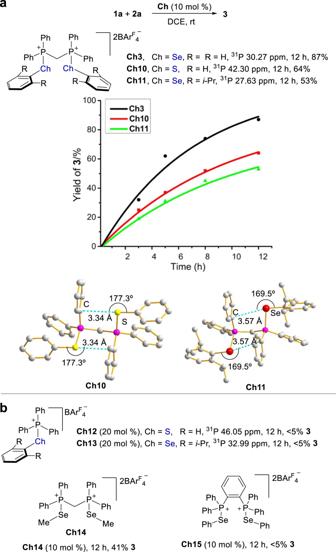Fig. 7: Structure and catalytic activity. aComparing the catalytic activity of analogous catalystsCh3,Ch10, andCh11.bCatalytic activity of reference catalystsCh12-15. 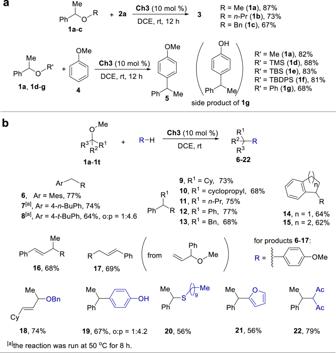Fig. 8: Chalcogen bonding catalytic transformation of ethers. aAlkoxide leaving groups.bCoupling reactions. 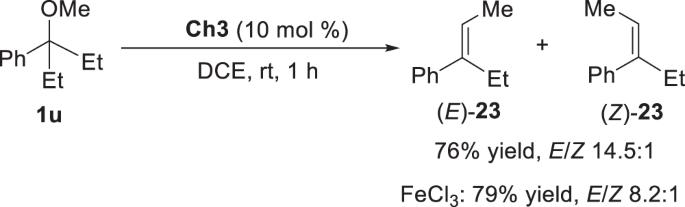Fig. 9: Stereospecific elimination. Chalcogen bonding catalysis approach to the elimination of ether 1u. The use of FeCl3as a reference Lewis acid catalyst for the elimination of ether 1u. 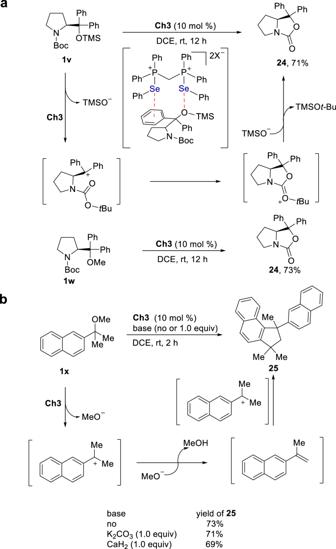Fig. 10: Cyclization of ethers. aIntramolecular cyclization reactions of1vand1w.bIntermolecular cyclization reaction of1x. Then the solvent was removed under reduced pressure, and the residue was purified by flash chromatography on silica gel to give the desired products.